Orphan receptor IL-17RD regulates Toll-like receptor signalling via SEFIR/TIR interactions Receptor families of the innate immune response engage in ‘cross-talk’ to tailor optimal immune responses against invading pathogens. However, these responses are subject to multiple levels of regulation to keep in check aberrant inflammatory signals. Here, we describe a role for the orphan receptor interleukin-17 receptor D (IL-17RD) in negatively regulating Toll-like receptor (TLR)-induced responses. Deficiency of IL-17RD expression in cells leads to enhanced pro-inflammatory signalling and gene expression in response to TLR stimulation, and Il17rd −/− mice are more susceptible to TLR-induced septic shock. We demonstrate that the intracellular Sef/IL-17R (SEFIR) domain of IL-17RD targets TIR adaptor proteins to inhibit TLR downstream signalling thus revealing a paradigm involving cross-regulation of members of the IL-17R and TLR families. The innate immune system has evolved a panoply of pattern-recognition receptors, including the transmembrane TLR family, to detect infection by recognizing highly conserved pathogen-associated molecular patterns, that are not found on host cells [1] . TLRs contain extracellular leucine-rich repeats that are integral in pathogen-associated molecular pattern binding, and a highly conserved intracellular domain that is shared with the interleukin (IL)-1 receptor family, the Toll/interleukin-1 receptor (TIR) domain [2] , [3] . The TIR domain is critical for recruiting one or more TIR-containing adaptor proteins to the plasma membrane to initiate downstream signalling pathways, resulting in activation of mitogen-activated protein kinases (MAPKs), NF-κB and interferon regulatory factors (IRFs), which promote transcription of pro-inflammatory genes. MyD88, the first TIR domain-containing adaptor to be characterized, is universally recruited by the IL-1 receptor family and all TLRs, except TLR3, for NF-κB activation [4] . MyD88-deficient mice still possess the ability to activate NF-κB, albeit with delayed kinetics, in response to lipopolysaccharide (LPS) and synthetic double-stranded RNA polyinosinic–polycytidylic acid (poly(I:C)), ligands for TLR4 and TLR3, respectively, indicating the existence of a MyD88-independent pathway for these receptors [5] , [6] , [7] . The discovery of Mal (or TIRAP) revealed that TLR2 and TLR4 bind MyD88 by employing Mal as a bridging adaptor [8] , [9] , [10] , [11] . Searches of the human genome for other TIR-containing proteins unveiled three more adaptors: TRIF, TRAM and SARM [12] , [13] , [14] . TRIF was revealed to be the adaptor utilized by TLR3 in NF-κB and IRF signalling [12] . TRIF is engaged directly by TLR3, but TLR4 requires a bridging adaptor and signals through TRIF by interacting primarily with TRAM [14] , [15] , [16] , [17] . SARM fails to activate NF-κB or IRF3 and has been described as a specific inhibitor of TRIF-dependent signalling [18] , [19] . MyD88 can activate downstream NF-κB and MAPK pathways by recruiting IRAK family members, which facilitate activation of the E3 ubiquitin ligase TRAF6 (refs 20 , 21 , 22 ). Formation of polyubiquination chains by TRAF6 acts as a platform for TAK1 to interact with its target substrates, the IκB kinases (IKKs), which subsequently phosphorylate the NF-κB inhibitor, IκB, leading to its proteasomal degradation and the subsequent release of NF-κB to the nucleus, where it activates transcription of pro-inflammatory genes [23] . TRAF6 also associates with TRIF and mediates NF-κB activation, although some reports suggest that RIP1 kinase is more important for this process [24] , [25] , [26] , [27] , [28] . TRIF also triggers IRF3 and IRF7 activation via the non-canonical IKK kinases, IKKi and TBK1, which phosphorylate IRF3 and IRF7 on serine residues, leading to their translocation to the nucleus and induction of type-I interferons (IFNs) [29] , [30] . Of increasing importance to the tailoring of innate immune responses initiated by TLRs, is the ability of innate immune signalling pathways to engage in ‘cross-talk’ to promote optimal immune responses. Recently, it was reported that the Sef/IL-17R (SEFIR) domains of the IL-17 receptors and the TIR domain of TLRs (which constitute a STIR domain superfamily) share similarity in length and secondary structure, especially in highly conserved boxes 1 and 2 of the TIR domain [31] . However, to date no data have been presented to implicate a functional interaction of these related domains. We have recently characterized the function of the orphan IL-17 receptor D (IL-17RD) in differentially regulating IL-17A-induced NF-κB and MAPK pathways [32] . The Il17rd gene encodes a transmembrane protein of the IL-17 receptor family, but its ligand remains unidentified [33] . IL-17RD, originally termed similar expression to fibroblast growth factor ( fgf ) genes (Sef) as it belonged to the FGF synexpression group in zebrafish development [34] , [35] , was initially established as a negative regulator of FGF-induced Ras and MAPK signalling pathways in zebrafish, and subsequently mammalian IL-17RD was reported to inhibit ERK and PI3K pathways in response to a number of receptor tyrosine kinase ligands [36] , [37] , [38] , [39] , [40] , [41] . We now show that IL-17RD is a negative regulator of both NF-κB and IRF signalling pathways initiated by TLRs. The SEFIR domain of IL-17RD targets the TIR adaptors, MyD88, Mal, TRIF and TRAM, and strongly inhibits TLR-mediated activation of NF-κB with IL-17RD deficiency leading to increased NF-κB and IRF activation and upregulation of pro-inflammatory genes. Il17rd −/− mice are more susceptible to TLR4- and TLR3-induced septic shock. We also present evidence for an autoregulatory feedback system in which IL-17RD targets TIR adaptors in a TLR stimulation-dependent manner thus precluding recruitment of the downstream effector TRAF6 and limiting pro-inflammatory gene expression. These findings describe a new regulatory network involving the functional interplay of members of the IL-17R and TLR families. IL-17RD inhibits TLR-induced signalling and gene expression Most TIR and SEFIR domain-containing proteins have the ability to trigger the activation of NF-κB. However, whereas the TIR adaptor proteins MyD88, Mal, TRIF and TRAM were capable of inducing an NF-κB-regulated luciferase reporter plasmid in HEK293 cells, overexpression of IL-17RD was ineffective ( Supplementary Fig. 1a ). In addition, overexpression of IL-17RD failed to induce IRF3 ( Supplementary Fig. 1b ) and IRF7 ( Supplementary Fig. 1c ) activation, unlike the upstream regulators IKKi and TBK1. Given the lack of effect of IL-17RD, we next probed its potential regulatory effects on TLR signalling. Co-transfection of cells with IL-17RD caused a dose-dependent inhibition of MyD88-, Mal-, TRIF- and TRAM-mediated induction of NF-κB-regulated luciferase ( Fig. 1a ). IL-17RD was also capable of inhibiting TRIF-induced expression of IRF3- and IRF7-regulated luciferase ( Fig. 1b ). We next explored the regulatory effects of IL-17RD on the induction of NF-κB and IRF-responsive genes. MyD88, Mal, TRIF and TRAM induced high levels of IL-8 production and this induction was inhibited by IL-17RD in a dose-dependent manner ( Fig. 1c ). TRIF induction of RANTES expression was also diminished in the presence of IL-17RD ( Fig. 1d ). To further explore the role of endogenous IL-17RD in TLR signalling, Il17rd gene expression was silenced by IL-17RD-specific small interfering RNA (siRNA) (previously described [32] ; Supplementary Fig. 1d , inset). Silencing of Il17rd gene expression in HEK293 cells resulted in augmented NF-κB activation in response to LPS and poly(I:C), while a scrambled control siRNA had no effect ( Supplementary Fig. 1d ). To validate these findings in other cell types, we established U373 and THP-1 cell lines that were selected for stable integration of lentivirus encoding IL-17RD-specific short hairpin RNA (shRNA) or control shRNA. Forty to sixty percent knockdown of Il17rd gene expression was consistently observed in U373 and THP-1 stable cell lines ( Supplementary Fig. 1f ). Knockdown of IL-17RD expression resulted in enhanced tumour necrosis factor-α (TNF-α) and IL-8 production in response to LPS, in U373 and THP-1 cells, respectively ( Fig. 1e,f ), and augmented poly(I:C)-induced RANTES and IP-10 production in U373 cells ( Fig. 1g ). This effect was mediated by increased gene expression, as LPS and poly(I:C) induced greater amounts of Il8 and Ifnb1 messenger RNA (mRNA) in THP-1 and U373 cells, respectively, stably expressing IL-17RD-specific shRNA ( Supplementary Fig. 1g,h ). These findings indicated that IL-17RD negatively regulates the expression of TLR3- and TLR4-responsive genes. This was further validated in human primary cells. Peripheral blood mononuclear cells (PBMCs) were isolated from blood of healthy volunteers and transfected with IL-17RD-specific and scrambled siRNAs. Knockdown of Il17rd gene expression in PBMCs ( Supplementary Fig. 1i ) augmented LPS- and poly(I:C)-induced expression of IL-8 and IFN-β production ( Supplementary Fig. 1j ). Given that IL-17RD regulated the levels of gene transcription, we next assessed its effects on the upstream signalling pathways that regulate such gene expression. Knockdown of IL-17RD in THP-1 cells ( Fig. 1h , inset panel) resulted in enhanced LPS-induced phosphorylation of IκBα and IKKs in response to LPS ( Fig. 1h ). Poly(I:C)-induced phosphorylation of IRF3 and its upstream kinase TBK1 was also accelerated and augmented in U373 cells expressing IL-17RD-specific shRNA compared with control cells ( Fig. 1i ), indicating that IL-17RD targets upstream regulators in these signal transduction pathways. 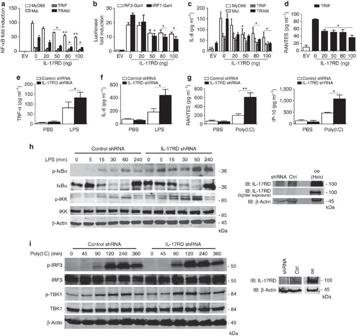Figure 1: IL-17RD negatively regulates TLR signalling pathways. (a,b) Assay of NF-κB-regulated luciferase reporter activity in HEK293 cells transfected with Myc-tagged IL-17RD (0–100 ng) and (a) MyD88, Mal, TRIF or TRAM (50 ng) with a NF-κB luciferase reporter plasmid (60 ng) or (b) with TRIF (50 ng) and PFR-luciferase (60 ng) with IRF3-Gal4 (30 ng) or IRF7-Gal4 (25 ng) constructs. TK Renilla was measured to determine transfection efficiency. (c,d) Supernatants were measured for (c) IL-8 or (d) RANTES production by sandwich ELISA. (e,f) ELISA of (e) TNF-α or (f) IL-8 from U373 or THP-1 cells, respectively, previously transduced with lentiviral-encoded control or IL-17RD-specific shRNA and treated with LPS (100 ng ml−1) for 24 h. (g) Supernatants from U373 cells stably transduced with control or IL-17RD-specific shRNA measured for RANTES and IP-10 levels by ELISA in response to poly(I:C) (25 μg ml−1). (h,i) Cell lysates from (h) THP-1 cells treated with LPS (100 ng ml−1) for 0, 5, 15, 30, 60 and 240 min and (i) U373 cells treated with poly(I:C) (25 μg ml−1) for 0, 45, 90, 120, 240 and 360 min, both stably expressing control and IL-17RD-specific shRNA, were subjected to immunoblotting with indicated antibodies. (h,i: inset panels) Cell lysates from THP-1 and U373 cells expressing control (Ctrl) or IL-17RD-specific shRNA (shRNA) were analysed for IL-17RD and β-actin expression with specific antibodies by immunoblotting. Overexpressed IL-17RD (oe) was used as a control from HEK293 and U373 cell lysates, respectively. Data are presented (a–g) as the mean ±s.e.m. of three independent experiments and were subjected to a two-tailed paired Student’st-test, *P<0.05; **P<0.01 or (h,i) are representative of three independent experiments. Images have been cropped for presentation. Full-size images are presented inSupplementary Fig. 7. Figure 1: IL-17RD negatively regulates TLR signalling pathways. ( a , b ) Assay of NF-κB-regulated luciferase reporter activity in HEK293 cells transfected with Myc-tagged IL-17RD (0–100 ng) and ( a ) MyD88, Mal, TRIF or TRAM (50 ng) with a NF-κB luciferase reporter plasmid (60 ng) or ( b ) with TRIF (50 ng) and PFR-luciferase (60 ng) with IRF3-Gal4 (30 ng) or IRF7-Gal4 (25 ng) constructs. TK Renilla was measured to determine transfection efficiency. ( c , d ) Supernatants were measured for ( c ) IL-8 or ( d ) RANTES production by sandwich ELISA. ( e , f ) ELISA of ( e ) TNF-α or ( f ) IL-8 from U373 or THP-1 cells, respectively, previously transduced with lentiviral-encoded control or IL-17RD-specific shRNA and treated with LPS (100 ng ml −1 ) for 24 h. ( g ) Supernatants from U373 cells stably transduced with control or IL-17RD-specific shRNA measured for RANTES and IP-10 levels by ELISA in response to poly(I:C) (25 μg ml −1 ). ( h , i ) Cell lysates from ( h ) THP-1 cells treated with LPS (100 ng ml −1 ) for 0, 5, 15, 30, 60 and 240 min and ( i ) U373 cells treated with poly(I:C) (25 μg ml −1 ) for 0, 45, 90, 120, 240 and 360 min, both stably expressing control and IL-17RD-specific shRNA, were subjected to immunoblotting with indicated antibodies. ( h , i : inset panels) Cell lysates from THP-1 and U373 cells expressing control (Ctrl) or IL-17RD-specific shRNA (shRNA) were analysed for IL-17RD and β-actin expression with specific antibodies by immunoblotting. Overexpressed IL-17RD (oe) was used as a control from HEK293 and U373 cell lysates, respectively. Data are presented ( a – g ) as the mean ±s.e.m. of three independent experiments and were subjected to a two-tailed paired Student’s t -test, * P <0.05; ** P <0.01 or ( h , i ) are representative of three independent experiments. Images have been cropped for presentation. Full-size images are presented in Supplementary Fig. 7 . Full size image IL-17RD deficiency enhances cell responsiveness to TLRs The above overexpression and knockdown studies strongly suggest that IL-17RD is a negative regulator of TLR adaptor-induced signalling. To confirm the physiological relevance of such findings, bone marrow-derived macrophages (BMDMs) from wild-type and IL-17RD-deficient mice [32] were compared for their responsiveness with various TLR ligands. All of the TLR ligands induced IL-6 protein in wild-type BMDMs, but the levels of induction were further enhanced in IL-17RD-deficient cells ( Fig. 2a ). Similarly, the levels of LPS- and poly(I:C)-induced RANTES ( Fig. 2b ) and poly(I:C)-induced IFN-β production ( Fig. 2c ) were greater in Il17rd −/− macrophages. Given the enhanced expression of TLR-responsive genes in IL-17RD-deficient cells, we were keen to assess gene expression in response to a live pathogen that triggers these pathways. 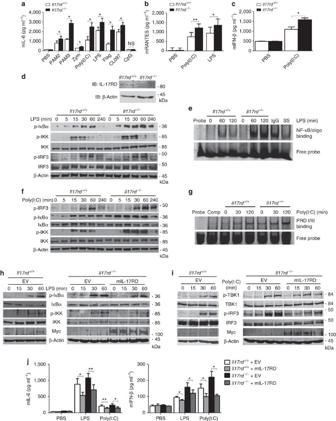Figure 2: IL-17RD deficiency enhances cell responsiveness to TLRs. (a–c) BMDMs from wild-type (WT) andIl17rd−/−mice were stimulated with (a) Pam2Cys (100 ng ml−1), Pam3Cys (100 ng ml−1), Zymosan (1 μg ml−1), poly(I:C) (5 μg ml−1), LPS (10 ng ml−1), CL097 (1 μg ml−1) and CpG (5 μg ml−1), (b) poly(I:C) (5 μg ml−1) and LPS (10 ng ml−1) for 24 h or (c) poly(I:C) (5 μg ml−1) for 24 h. Conditioned media was assayed for (a) IL-6, (b) RANTES or (c) IFN-β. (d,f) WT andIl17rd−/−BMDMs were treated with (d) LPS (10 ng ml−1) or (f) poly(I:C) (5 μg ml−1) for 0–240 min and cell lysates immunoblotted with indicated antibodies. (d, inset panel) Cell lysates from WT andIl17rd−/−BMDCs were immunoblotted for IL-17RD and β-actin expression. (e) WT andIl17rd−/−BMDMs were stimulated with LPS (10 ng ml−1) for 0–120 min and nuclear extracts assayed by EMSA for NF-κB/DNA binding. Nuclear extracts (fromIl17rd−/−cells stimulated with LPS for 60 min) were also pre-incubated for 15 min with 1 μg anti-p65 antibody (ss; supershift) or IgG control (IgG). (g) WT andIl17rd−/−BMDCs were stimulated with poly(I:C) (5 μg ml−1) for 0–120 min and nuclear extracts assayed by EMSA using an oligonucleotide containing the PRD I/III domain of theIfnb1promoter. Nuclear extracts (fromIl17rd−/−cells stimulated with poly(I:C) for 30 min) were also pre-incubated for 15 min with an unlabelled competitor oligonucleotide. (h–j) WT andIl17rd−/−MEFs were infected with MSCV retroviral particles containing an empty vector (EV) plasmid or wild-type mIL-17RD-Myc (Il17rd−/−MEFs) for 72 h. Cells were treated with (h) LPS (100 ng ml−1) or (i) poly(I:C) (25 μg ml−1) for 0–60 min and cell lysates immunoblotted with indicated antibodies or cells were treated with (j) LPS (100 ng ml−1) or poly(I:C) (25 μg ml−1) for 24 h and conditioned media assayed for levels of IL-6 and IFN-β. Data are presented (a–c,j) as the mean ±s.e.m. of three independent experiments and were subjected to a two-tailed paired Student’st-test, *P<0.05; **P<0.01 or (d–i) are representative of three independent experiments. Images have been cropped for presentation. Full-size images are presented inSupplementary Fig. 8. NS, not significant. Figure 2: IL-17RD deficiency enhances cell responsiveness to TLRs. ( a – c ) BMDMs from wild-type (WT) and Il17rd −/− mice were stimulated with ( a ) Pam2Cys (100 ng ml −1 ), Pam3Cys (100 ng ml −1 ), Zymosan (1 μg ml −1 ), poly(I:C) (5 μg ml −1 ), LPS (10 ng ml −1 ), CL097 (1 μg ml −1 ) and CpG (5 μg ml −1 ), ( b ) poly(I:C) (5 μg ml −1 ) and LPS (10 ng ml −1 ) for 24 h or ( c ) poly(I:C) (5 μg ml −1 ) for 24 h. Conditioned media was assayed for ( a ) IL-6, ( b ) RANTES or ( c ) IFN-β. ( d , f ) WT and Il17rd −/− BMDMs were treated with ( d ) LPS (10 ng ml −1 ) or ( f ) poly(I:C) (5 μg ml −1 ) for 0–240 min and cell lysates immunoblotted with indicated antibodies. ( d , inset panel) Cell lysates from WT and Il17rd −/− BMDCs were immunoblotted for IL-17RD and β-actin expression. ( e ) WT and Il17rd −/− BMDMs were stimulated with LPS (10 ng ml −1 ) for 0–120 min and nuclear extracts assayed by EMSA for NF-κB/DNA binding. Nuclear extracts (from Il17rd −/− cells stimulated with LPS for 60 min) were also pre-incubated for 15 min with 1 μg anti-p65 antibody (ss; supershift) or IgG control (IgG). ( g ) WT and Il17rd −/− BMDCs were stimulated with poly(I:C) (5 μg ml −1 ) for 0–120 min and nuclear extracts assayed by EMSA using an oligonucleotide containing the PRD I/III domain of the Ifnb1 promoter. Nuclear extracts (from Il17rd −/− cells stimulated with poly(I:C) for 30 min) were also pre-incubated for 15 min with an unlabelled competitor oligonucleotide. ( h – j ) WT and Il17rd −/− MEFs were infected with MSCV retroviral particles containing an empty vector (EV) plasmid or wild-type mIL-17RD-Myc ( Il17rd −/− MEFs) for 72 h. Cells were treated with ( h ) LPS (100 ng ml −1 ) or ( i ) poly(I:C) (25 μg ml −1 ) for 0–60 min and cell lysates immunoblotted with indicated antibodies or cells were treated with ( j ) LPS (100 ng ml −1 ) or poly(I:C) (25 μg ml −1 ) for 24 h and conditioned media assayed for levels of IL-6 and IFN-β. Data are presented ( a – c , j ) as the mean ±s.e.m. of three independent experiments and were subjected to a two-tailed paired Student’s t -test, * P <0.05; ** P <0.01 or ( d – i ) are representative of three independent experiments. Images have been cropped for presentation. Full-size images are presented in Supplementary Fig. 8 . NS, not significant. Full size image Murine embryonic fibroblasts (MEFs) from wild-type and Il17rd −/− embryos were infected with encephalomyocarditis virus (EMCV) and expression levels of pro-inflammatory cytokines and chemokines were measured. EMCV induced IL-6, KC and RANTES production in wild-type MEFs, but levels of induction were greater in IL-17RD-deficient cells ( Supplementary Fig. 2a ). The greater expression of TLR- and EMCV-responsive genes in IL-17RD-deficient cells seems to be due to regulatory effects on gene transcription as indicated by enhanced LPS-induced expression of Cxcl1 and Il6 mRNAs ( Supplementary Fig. 2b ) and EMCV-induced Ifnb1 mRNA in Il17rd −/− cells relative to wild-type counterparts ( Supplementary Fig. 2c ). Given that the effects of IL-17RD deficiency on TLR-responsive gene expression manifest as changes in their levels of transcription, we next characterized the upstream signalling pathways that regulates such transcription. LPS-induced phosphorylation of IκBα, IKK and IRF3 was accelerated and more pronounced in IL-17RD-deficient BMDMs compared with wild-type cells ( Fig. 2d ), suggesting that loss of IL-17RD leads to greater activation of NF-κB and IRF3. This was confirmed by electromobility-shift assays (EMSAs) in which nuclear extracts from LPS-stimulated Il17rd −/− BMDMs ( Fig. 2e ) and Il17rd −/− MEFs ( Supplementary Fig. 2d ) showed more binding, than extracts from corresponding wild-type cells, to an oligonucleotide containing the NF-κB recognition motif. The enhanced activation of NF-κB and IRF3 in the absence of IL-17RD also extended to the TLR3 pathway, since poly(I:C)-mediated phosphorylation of IRF3, IκBα and IKKs ( Fig. 2f ) and IRF3/IRF7 binding to the enhancer region of the Ifnb1 gene ( Fig. 2g ) were more intense in Il17rd −/− cells relative to wild-type cells. Given that IL-17RD was initially characterized as a negative regulator of FGF-induced ERK signalling, we also assessed the effects of IL-17RD deficiency on activation of the ERK pathway in response to LPS. Under these conditions, the levels of ERK phosphorylation were increased basally and in LPS-stimulated IL-17RD-deficient MEFs ( Supplementary Fig. 3a ) and bone marrow-derived dendritic cells (BMDCs) ( Supplementary Fig. 3b ), suggesting that IL-17RD negatively regulates LPS-induced activation of ERKs. To validate that enhanced TLR responses in cells lacking IL-17RD are directly attributable to loss of IL-17RD expression, we transduced IL-17RD-deficient MEFs with retrovirus encoding murine Myc-tagged IL-17RD or an empty vector. Reconstitution of Il17rd −/− MEFs with mIL-17RD reduced LPS-induced phosphorylation of IκBα and IKKs ( Fig. 2h ) and poly(I:C)-induced phosphorylation of TBK1 and IRF3 ( Fig. 2i ) to levels comparable to wild-type cells. Furthermore, reconstitution of cells with mIL-17RD also reduced the efficacy of LPS and poly(I:C) in driving expression of IL-6 and IFN-β ( Fig. 2j ). IL-17RD-deficient mice are more susceptible to septic shock The above cell-based approaches demonstrate that a loss of IL-17RD expression results in a heightened pro-inflammatory response to TLR ligands. We next investigated the in vivo relevance of such effects. Wild-type and Il17rd −/− mice were challenged with LPS by intraperitoneal (i.p.) injection and assessed for systemic inflammation. LPS induced lethality in 37% of wild-type mice, but this increased to 81% in the case of IL-17RD-deficient mice with death also being evident at earlier times post LPS administration ( Fig. 3a ). Lower resistance of Il17rd −/− mice to TLR4-induced septic shock correlated with significantly increased serum concentrations of IL-6, KC and the IL-12/IL-23 p40 subunit in IL-17RD-deficient mice challenged with LPS for 16 h compared with wild-type mice ( Fig. 3b ). Transcription of the genes encoding inducible nitric oxide synthase (iNOS), TNF-α and IL-6 were also substantially upregulated in the spleen of Il17rd −/− mice compared with wild-type mice in response to LPS ( Fig. 3c ). To determine whether Il17rd −/− mice were also more susceptible to TLR3-induced death, mice were subjected to i.p. injection of poly(I:C) co-administered with a liver-specific transcription inhibitor, D -galactosamine ( D -GAL), to enhance toxicity [42] ( Fig. 3d ). A low dose of poly(I:C) with D -GAL induced death in less than 20% of wild-type mice in 24 h; however, 50% of Il17rd −/− mice succumbed to poly(I:C)-induced death. Examination of liver tissue from surviving poly(I:C)-treated wild-type mice by microscopy revealed histopathological changes with normal liver architecture, mild hepatocyte vacuolation and occasional individual necrotic cells ( Fig. 3e ). In contrast, surviving Il17rd −/− mice showed distorted liver architecture due to widespread areas of necrosis, characterized by pyknotic nuclei, with pooling of red blood cells from the sinuses. Consistent with lethality results, serum concentrations of IFN-β, RANTES, IL-6 and the IL-12/IL-23 p40 subunit were greatly augmented in Il17rd −/− mice compared with wild-type mice after 16 h of poly(I:C) challenge ( Fig. 3f ). The enhanced type-I IFN in serum of Il17rd −/− mice was bioactive ( Fig. 3g ). Poly(I:C)-mediated transcription of Cxcl10 and Ccl5 genes were also increased in spleens from Il17rd −/− mice compared with wild-type mice ( Fig. 3h ). Overall these findings provide strong support for a physiological role for IL-17RD in negatively regulating the host response to stimulation of TLR3 and TLR4. 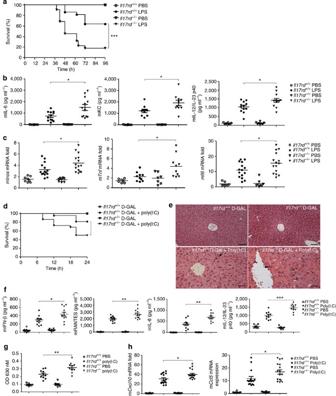Figure 3:Il17rd−/−mice are more susceptible to TLR-induced lethality. (a) Survival of age- and sex-matched WT andIl17rd−/−mice (n=22) injected i.p. with LPS (20 mg per kg body weight) over 96 h. (b) Sandwich ELISA of IL-6, KC and the IL-12/IL-23 p40 subunit in serum of age- and sex-matched WT andIl17rd−/−mice (n=10–12) measured 16 h after i.p. injection with LPS (20 mg kg−1). (c) Quantitative PCR (qPCR) analysis ofInos,TnfandIl6mRNA levels in spleens from WT andIl17rd−/−mice (n=10–15) 16 h after i.p. injection with LPS. (d) Survival of age- and sex-matched WT andIl17rd−/−mice (n=22) injected i.p. with poly(I:C) (0.01 μg per g body weight) andD-galactosamine (0.7 mg per g body weight) over 24 h. (e) Representative images of haematoxylin and eosin staining of liver from surviving WT andIl17rd−/−mice injected i.p. with poly(I:C) andD-galactosamine. Images were captured at magnifications of × 20 (upper panels: scale bar, 100 μm) and × 40 (lower panels: scale bar, 50 μm). (f) Serum of age- and sex-matched WT andIl17rd−/−mice (n=10–12) after i.p. injection with poly(I:C) (5 mg per kg body weight) for 16 h was measured for IFN-β, RANTES, IL-6 and the IL-12/IL-23 p40 subunit levels by ELISA. (g) Expression of bioactive type-I interferon was measured by blue sensor cells. (h) qPCR analysis ofCxcl10andCcl5mRNA levels in spleen samples from WT andIl17rd−/−mice (n=16) 16 h after i.p. injection with poly(I:C) (5 mg kg−1). Data are (e) representative ofn=9, or presented (b,c,f–h) as the mean ±s.e.m. of three independent experiments and were subjected to a two-tailed unpaired Student’st-test, *P<0.05; **P<0.01; ***P<0.001, or (a,d) the log-rank test (PBS/D-GALn=10) (LPS/poly(I:C)n=22). Figure 3: Il17rd −/− mice are more susceptible to TLR-induced lethality. ( a ) Survival of age- and sex-matched WT and Il17rd −/− mice ( n =22) injected i.p. with LPS (20 mg per kg body weight) over 96 h. ( b ) Sandwich ELISA of IL-6, KC and the IL-12/IL-23 p40 subunit in serum of age- and sex-matched WT and Il17rd −/− mice ( n =10–12) measured 16 h after i.p. injection with LPS (20 mg kg −1 ). ( c ) Quantitative PCR (qPCR) analysis of Inos , Tnf and Il6 mRNA levels in spleens from WT and Il17rd −/− mice ( n =10–15) 16 h after i.p. injection with LPS. ( d ) Survival of age- and sex-matched WT and Il17rd −/− mice ( n =22) injected i.p. with poly(I:C) (0.01 μg per g body weight) and D -galactosamine (0.7 mg per g body weight) over 24 h. ( e ) Representative images of haematoxylin and eosin staining of liver from surviving WT and Il17rd −/− mice injected i.p. with poly(I:C) and D -galactosamine. Images were captured at magnifications of × 20 (upper panels: scale bar, 100 μm) and × 40 (lower panels: scale bar, 50 μm). ( f ) Serum of age- and sex-matched WT and Il17rd −/− mice ( n =10–12) after i.p. injection with poly(I:C) (5 mg per kg body weight) for 16 h was measured for IFN-β, RANTES, IL-6 and the IL-12/IL-23 p40 subunit levels by ELISA. ( g ) Expression of bioactive type-I interferon was measured by blue sensor cells. ( h ) qPCR analysis of Cxcl10 and Ccl5 mRNA levels in spleen samples from WT and Il17rd −/− mice ( n =16) 16 h after i.p. injection with poly(I:C) (5 mg kg −1 ). Data are ( e ) representative of n =9, or presented ( b , c , f – h ) as the mean ±s.e.m. of three independent experiments and were subjected to a two-tailed unpaired Student’s t -test, * P <0.05; ** P <0.01; *** P <0.001, or ( a , d ) the log-rank test (PBS/D-GAL n =10) (LPS/poly(I:C) n =22). Full size image SEFIR domain is critical for inhibitory effects of IL-17RD The important regulatory role of IL-17RD in dampening the TLR-induced inflammatory response prompted studies on the mechanism by which IL-17RD exerts its inhibitory function. Given that IL-17RD contains a SEFIR domain, which shares some structural similarity with the TIR domain [31] , and our earlier observations that IL-17RD inhibits signalling downstream of TIR adaptors, we examined whether IL-17RD could target TIR adaptors as part of their inhibitory function. Co-immunoprecipitation analysis demonstrated that IL-17RD can interact with co-expressed MyD88 or Mal ( Fig. 4a ). The ability of IL-17RD to interact with these TIR adaptors was further supported by confocal microscopy revealing co-localization of IL-17RD and MyD88 in cytoplasmic vesicle structures ( Fig. 4b ). We next investigated whether the SEFIR domain was required for this interaction. A truncation mutant of IL-17RD lacking the C-terminal SEFIR domain, termed IL-17RDΔC, was thus generated ( Supplementary Fig. 4a ) and assessed for ability to interact with MyD88 by co-immunoprecipitation analysis. Unlike full-length IL-17RD, IL-17RDΔC failed to show any detectable interaction with MyD88 ( Fig. 4c ). Furthermore, IL-17RDΔC was unable to inhibit MyD88-activation of NF-κB ( Fig. 4d ), suggesting that the interaction of IL-17RD with TIR adaptors and its inhibitory effects are SEFIR domain dependent. Since TLR4 and TLR3 also each contain a TIR domain, we also demonstrated that IL-17RD interacts with TLR4 ( Fig. 4e ) and TLR3 ( Supplementary Fig. 4b ) in a SEFIR domain-dependent manner. We next examined whether the SEFIR domain alone of IL-17RD was sufficient to interact with the TIR domain and manifest its inhibitory effects. A mutant encoding only the IL-17RD SEFIR domain was thus generated and termed IL-17RD SEFIR ( Supplementary Fig. 4a ). The IL-17RD SEFIR domain was capable of interacting with MyD88 ( Fig. 4f ) and like the full-length IL-17RD was also capable of interacting with other TIR adaptors including Mal and TRIF, while IL-17RDΔC, lacking the SEFIR domain, failed to do so ( Supplementary Fig. 4c,d ). Intriguingly, the IL-17RD SEFIR domain was unable to interact with TLR4 ( Fig. 4g ) and TLR3 ( Supplementary Fig. 4e ), suggesting that the SEFIR domain of IL-17RD is not sufficient for mediating binding to TIR domain-containing TLRs. However, the IL-17RD SEFIR was sufficient to effect a dose-dependent inhibition of MyD88-mediated NF-κB activation ( Fig. 4h ). Given these inhibitory effects of the SEFIR domain of IL-17RD, we were keen to assess whether other SEFIR domain-containing proteins, such as IL-17RA and Act1, could similarly inhibit MyD88-induced activation of NF-κB. The expression of full-length IL-17RA and Act1 or their SEFIR domains failed to affect MyD88-induced NF-κB activation ( Supplementary Fig. 4f ), suggesting that the inhibitory effects are restricted to the IL-17RD-SEFIR domain. In addition to the SEFIR domain, IL-17RD contains a putative TRAF6-binding site (PRERL; residues 348–352) that is positioned immediately upstream of the SEFIR domain [39] . Mutation of the conserved glutamic-acid residue (E350A) failed to affect the ability of IL-17RD to inhibit MyD88-induced NF-κB activation ( Supplementary Fig. 4g ) or to interact with MyD88 ( Supplementary Fig. 4h ). Interestingly, tyrosine residue 330 in IL-17RD had previously been described as indispensable for the regulatory effects of IL-17RD on FGF signalling [43] . Given that this residue also lies in close proximity to the IL-17RD-SEFIR domain, we also assessed the regulatory effects of a point mutant form of IL-17RD in which this tyrosine residue was mutated to phenylalanine. The point mutant form mimicked wild-type IL-17RD in its inhibitory effects on MyD88-induced NF-κB activation ( Supplementary Fig. 4i ) and retained the ability of wild-type IL-17RD to interact with MyD88 ( Supplementary Fig. 4j ), indicating that IL-17RD regulates FGF and TLR signalling by distinct mechanisms. In relation to TLR signalling, the above data collectively indicate that the IL-17RD-SEFIR domain targets TLR pathways at the level of TIR adaptor proteins to inhibit downstream TLR signalling. 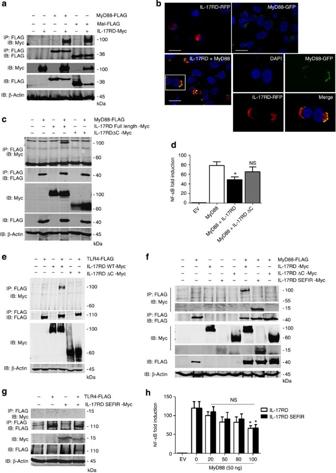Figure 4: SEFIR domain is critical for inhibitory effects of IL-17RD. (a) HEK293 cells were transfected for 24 h with (a) MyD88-FLAG, Mal-FLAG and IL-17RD-Myc (1 μg). Cell lysates were immunoprecipitated with an anti-FLAG antibody, followed by immunoblotting with indicated antibodies. (b) HEK293 cells were transfected for 24 h with MyD88-GFP and IL-17RD-RFP and visualized for expression and localization using confocal microscopy. Cells were also incubated with nuclei-staining DAPI. Confocal images were captured using the × 63 objective (oil immersion) on the UV Zeiss 510 Meta System laser scanning microscope equipped with the appropriate filter sets and analysed using the LSM 5 browser imaging software (scale bar, 20 μm). (c) HEK293 cells were transfected for 24 h with MyD88-FLAG with IL-17RD-Myc or IL-17RD ΔC-Myc (1 μg). Cell lysates were immunoprecipitated with an anti-FLAG antibody, followed by immunoblotting with indicated antibodies. (d) Assay of NF-κB-regulated luciferase expression in HEK293 cells transfected with MyD88 (50 ng) with IL-17RD-Myc or IL-17RD ΔC-Myc (50 ng). (e–g) HEK293 cells were transfected for 24 h with (e) TLR4-FLAG and IL-17RD-Myc or IL-17RD ΔC-Myc, (f) MyD88-FLAG and IL-17RD-Myc, IL-17RD ΔC-Myc and IL-17RD SEFIR-Myc or (g) TLR4-FLAG and IL-17RD SEFIR-Myc (1 μg). Cell lysates were immunoprecipitated with an anti-FLAG antibody, followed by immunoblotting with indicated antibodies. (h) Assay of NF-κB regulated luciferase expression in HEK293 cells transfected with MyD88 (50 ng) and IL-17RD-Myc or IL-17RD SEFIR-Myc (100 ng). Data are (a–c,e–g) representative of three independent experiments or (d,h) are presented as the mean ±s.e.m. of three independent experiments and were subjected to a two-tailed paired Student’st-test. *P<0.05. Images have been cropped for presentation. Full-size images are presented inSupplementary Fig. 9. NS, not significant. Figure 4: SEFIR domain is critical for inhibitory effects of IL-17RD. ( a ) HEK293 cells were transfected for 24 h with ( a ) MyD88-FLAG, Mal-FLAG and IL-17RD-Myc (1 μg). Cell lysates were immunoprecipitated with an anti-FLAG antibody, followed by immunoblotting with indicated antibodies. ( b ) HEK293 cells were transfected for 24 h with MyD88-GFP and IL-17RD-RFP and visualized for expression and localization using confocal microscopy. Cells were also incubated with nuclei-staining DAPI. Confocal images were captured using the × 63 objective (oil immersion) on the UV Zeiss 510 Meta System laser scanning microscope equipped with the appropriate filter sets and analysed using the LSM 5 browser imaging software (scale bar, 20 μm). ( c ) HEK293 cells were transfected for 24 h with MyD88-FLAG with IL-17RD-Myc or IL-17RD ΔC-Myc (1 μg). Cell lysates were immunoprecipitated with an anti-FLAG antibody, followed by immunoblotting with indicated antibodies. ( d ) Assay of NF-κB-regulated luciferase expression in HEK293 cells transfected with MyD88 (50 ng) with IL-17RD-Myc or IL-17RD ΔC-Myc (50 ng). ( e – g ) HEK293 cells were transfected for 24 h with ( e ) TLR4-FLAG and IL-17RD-Myc or IL-17RD ΔC-Myc, ( f ) MyD88-FLAG and IL-17RD-Myc, IL-17RD ΔC-Myc and IL-17RD SEFIR-Myc or ( g ) TLR4-FLAG and IL-17RD SEFIR-Myc (1 μg). Cell lysates were immunoprecipitated with an anti-FLAG antibody, followed by immunoblotting with indicated antibodies. ( h ) Assay of NF-κB regulated luciferase expression in HEK293 cells transfected with MyD88 (50 ng) and IL-17RD-Myc or IL-17RD SEFIR-Myc (100 ng). Data are ( a – c , e – g ) representative of three independent experiments or ( d , h ) are presented as the mean ±s.e.m. of three independent experiments and were subjected to a two-tailed paired Student’s t -test. * P <0.05. Images have been cropped for presentation. Full-size images are presented in Supplementary Fig. 9 . NS, not significant. Full size image IL-17RD disrupts signalling downstream of TIR adaptors We next investigated how the targeting of TIR adaptors by IL-17RD interfered with downstream signalling pathways. We were especially keen to assess whether IL-17RD affected the recruitment of TIR adaptors to TLRs and/or the interaction of adaptors with key downstream effector molecules such as TRAF6. Wild-type and Il17rd −/− BMDMs were treated with LPS, and lysates were immunoprecipitated for endogenous MyD88 and assessed for co-precipitated TLR4 and TRAF6. The loss of IL-17RD expression in Il17rd −/− BMDMs had little effect on the interaction of TLR4 with MyD88 in response to LPS ( Fig. 5a ). However, the LPS-induced recruitment of TRAF6 to the MyD88 signalling complex was augmented in IL-17RD-deficient cells ( Fig. 5a ), suggesting that IL-17RD tempers the ability of MyD88 to recruit downstream effector molecules. We investigated the functional consequence of this regulatory effect of IL-17RD by assessing polyubiquitination of TRAF6 in response to TLR4 stimulation. LPS induced a time-dependent polyubiquitination of TRAF6 in wild-type BMDMs but this was greatly enhanced in IL-17RD-deficient BMDMs ( Fig. 5b ), indicating that the regulatory effects of IL-17RD on MyD88–TRAF6 interaction results in decreased ubiquitination of TRAF6. Poly(I:C)-induced polyubiquitination of TRAF6 is also greatly augmented in IL-17RD-deficient cells ( Fig. 5c ), suggesting that IL-17RD targets the TLR signalling pathway at the level of TIR adaptors recruiting and activating downstream effectors. This model was further supported by the demonstration that IL-17RD directly inhibits the recruitment of TRAF6 to the MyD88 signalling complex ( Fig. 5d ). Interestingly, the IL-17RD SEFIR domain mutant is also capable of exerting such inhibitory effects, whereas the IL-17RD ΔC mutant, lacking the SEFIR domain, is ineffective ( Fig. 5d ). We next probed whether the IL-17RD-SEFIR domain recognizes the TIR domain of MyD88, and to this end we generated a truncated mutant (amino acids 160–296) constituting the TIR domain of MyD88. The IL-17RD-SEFIR domain mutant was capable of interacting with MyD88 TIR ( Supplementary Fig. 5a ) and the interaction of MyD88 TIR with TRAF6 was reduced with co-expression of IL-17RD SEFIR ( Supplementary Fig. 5b ), suggesting that IL-17RD SEFIR targets the TIR domain of MyD88. IL-17RA, Act1 and their SEFIR domains were also assessed for their ability to disrupt the MyD88/TRAF6 signalling complex. IL-17RA and the SEFIR domains of IL-17RA and Act1 failed to replicate the ability of IL-17RD to disrupt the MyD88/TRAF6 interaction ( Supplementary Fig. 5c ) and this is consistent with our earlier data above demonstrating the specific inhibitory effects of IL-17RD and its SEFIR domain on MyD88-induced activation of NF-κB ( Supplementary Fig. 4f ). This supports a model in which the IL-17RD-SEFIR domain targets the TIR domain of MyD88 and inhibits downstream recruitment of TRAF6. Interestingly, overexpression of full-length Act1 inhibited the MyD88/TRAF6 interaction, but this is not mediated by its SEFIR domain ( Supplementary Fig. 5c ) and is more likely due to its previously characterized ability to bind to TRAF6 (ref. 44 ). It is possible that this might preclude binding of the latter to MyD88. 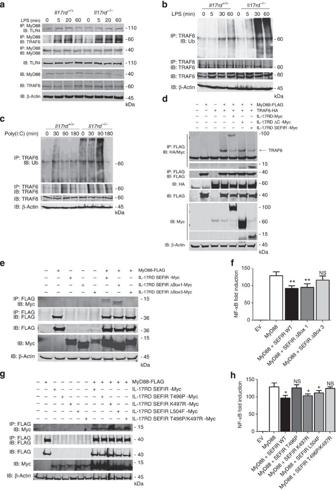Figure 5: IL-17RD disrupts signalling downstream of TIR adaptors. (a) WT andIl17rd−/−BMDMs were stimulated for 0, 5, 20 and 60 min with LPS (10 ng ml−1) and cell lysates were subject to immunoprecipitation with an anti-MyD88 antibody and subjected to immunoblotting with indicated antibodies. (b,c) WT andIl17rd−/−BMDMs or BMDCs were treated for (b) 0, 5, 30 and 60 min with LPS (10 ng ml−1) or (c) 0, 30, 90 and 180 min poly(I:C) (5 μg ml−1), respectively. Cell lysates were subject to SDS treatment, immunoprecipitation with an anti-TRAF6 antibody and probed by immunoblotting with indicated antibodies. (d,e,g) HEK293 cells were transfected for 24 h with MyD88-FLAG with (d) TRAF6-HA with IL-17RD-Myc, IL-17RD ΔC-Myc or IL-17RD SEFIR-Myc (total 3 μg) or (e) Myc-tagged IL-17RD SEFIR, IL-17RD SEFIR ΔBox1 or IL-17RD SEFIR ΔBox3 or (g) Myc-tagged IL-17RD SEFIR, IL-17RD SEFIR T496P, IL-17RD SEFIR K497R, IL-17RD SEFIR L504F or IL-17RD SEFIR T496P/K497R. Cell lysates were immunoprecipitated with an anti-FLAG antibody, followed by immunoblotting with indicated antibodies. (f,h) Assay of NF-κB-regulated luciferase expression in HEK 293 cells transfected with MyD88 (50 ng) with (f) Myc-tagged IL-17RD SEFIR, IL-17RD SEFIR ΔBox1 or IL-17RD SEFIR ΔBox3 (100 ng) or (h) Myc-tagged IL-17RD SEFIR, IL-17RD SEFIR T496P, IL-17RD SEFIR K497R, IL-17RD SEFIR L504F or IL-17RD SEFIR T496P/K497R (100 ng). Data are (a–e,g) representative of three independent experiments or (f,h) are presented as the mean ±s.e.m. of three independent experiments and were subjected to a two-tailed paired Student’st-test. *P<0.05; **P<0.01. Images have been cropped for presentation. Full-size images are presented inSupplementary Fig. 10. NS, not significant. Figure 5: IL-17RD disrupts signalling downstream of TIR adaptors. ( a ) WT and Il17rd −/− BMDMs were stimulated for 0, 5, 20 and 60 min with LPS (10 ng ml −1 ) and cell lysates were subject to immunoprecipitation with an anti-MyD88 antibody and subjected to immunoblotting with indicated antibodies. ( b , c ) WT and Il17rd −/− BMDMs or BMDCs were treated for ( b ) 0, 5, 30 and 60 min with LPS (10 ng ml −1 ) or ( c ) 0, 30, 90 and 180 min poly(I:C) (5 μg ml −1 ), respectively. Cell lysates were subject to SDS treatment, immunoprecipitation with an anti-TRAF6 antibody and probed by immunoblotting with indicated antibodies. ( d , e , g ) HEK293 cells were transfected for 24 h with MyD88-FLAG with ( d ) TRAF6-HA with IL-17RD-Myc, IL-17RD ΔC-Myc or IL-17RD SEFIR-Myc (total 3 μg) or ( e ) Myc-tagged IL-17RD SEFIR, IL-17RD SEFIR ΔBox1 or IL-17RD SEFIR ΔBox3 or ( g ) Myc-tagged IL-17RD SEFIR, IL-17RD SEFIR T496P, IL-17RD SEFIR K497R, IL-17RD SEFIR L504F or IL-17RD SEFIR T496P/K497R. Cell lysates were immunoprecipitated with an anti-FLAG antibody, followed by immunoblotting with indicated antibodies. ( f , h ) Assay of NF-κB-regulated luciferase expression in HEK 293 cells transfected with MyD88 (50 ng) with ( f ) Myc-tagged IL-17RD SEFIR, IL-17RD SEFIR ΔBox1 or IL-17RD SEFIR ΔBox3 (100 ng) or ( h ) Myc-tagged IL-17RD SEFIR, IL-17RD SEFIR T496P, IL-17RD SEFIR K497R, IL-17RD SEFIR L504F or IL-17RD SEFIR T496P/K497R (100 ng). Data are ( a – e , g ) representative of three independent experiments or ( f , h ) are presented as the mean ±s.e.m. of three independent experiments and were subjected to a two-tailed paired Student’s t -test. * P <0.05; ** P <0.01. Images have been cropped for presentation. Full-size images are presented in Supplementary Fig. 10 . NS, not significant. Full size image We next probed the molecular basis to why the SEFIR domain of IL-17RD mediates inhibitory effects on MyD88 signalling, whereas other SEFIR domain-containing proteins such as IL-17RA are ineffective. A previous comparison analysis of TIR and SEFIR domains, using sequence alignments and secondary-structure predictions, indicated similarity between these domains [31] . The latter study also proposed that of the three box regions of the TIR domain, box 1 and box 2, but not box 3, are conserved in the SEFIR domain. Given that these box regions facilitate homotypic TIR interactions, we performed a simple sequence alignment (using ClustalW2 ( http://www.ebi.ac.uk/Tools/msa/clustalw2/ ) and BoxShade software ( http://www.ch.embnet.org/software/BOX_form.html ) of the TIR domain of MyD88 and the SEFIR domains of IL-17RA and IL-17RD to examine differences between IL-17RA and IL-17RD in these box regions. IL-17RA and IL-17RD showed sequence similarity in their regions corresponding to box 2 of MyD88 ( Supplementary Fig. 5d,e ), suggesting that these regions are unlikely to explain the differential effects of the SEFIR domain in IL-17RA and IL-17RD. However, there was more divergence in sequence between IL-17RA and IL-17RD in the regions corresponding to box 1 and 3 of MyD88, and to this end we generated truncation mutants of IL-17RD that lacked the box 1 (IL-17RD SEFIR ΔBox1) or the box 3 region (IL-17RD SEFIR ΔBox3) ( Supplementary Fig. 5e ). Like the full-length SEFIR domain of IL-17RD, the IL-17RD SEFIR ΔBox1 mutant was capable of interacting with MyD88, but the IL-17RD SEFIR ΔBox3 mutant failed to associate with MyD88 ( Fig. 5e ). In addition, the IL-17RD SEFIR ΔBox3 mutant failed to inhibit MyD88-induced NF-κB activation, whereas IL-17RD SEFIR and the IL-17RD SEFIR ΔBox1 mutant showed inhibitory effects ( Fig. 5f ). This demonstrates that the C-terminal region of the IL-17RD SEFIR domain, which is located at a position corresponding to box 3 of MyD88, is critical for the functional effects of IL-17RD in regulating MyD88-induced signalling pathways. We next attempted to identify critical individual amino-acid residues in the C-terminal region of the IL-17RD SEFIR. Intriguingly, the sequence alignment shows three amino-acid residues in this region of IL-17RD (T496, K497 and L504) that are also present in MyD88 but not in IL-17RA ( Supplementary Fig. 5d,e ). Each of these residues in the SEFIR domain of IL-17RD were mutated to the corresponding residues in IL-17RA (T496P, K497R and L504F) and a double mutation of the adjacent T496 and K497 residues was also performed (T496P/K497R). All four mutants retained the ability of the SEFIR domain of IL-17RD to associate with MyD88 ( Fig. 5g ), but interestingly the T496P and T496P/K497R mutants failed to inhibit MyD88-induced activation of NF-κB ( Fig. 5h ). These data indicate that the C-terminal region of the IL-17RD SEFIR domain is critical for its interaction with MyD88, and T496 is a key residue for manifesting its functional effects on MyD88 signalling. It is especially interesting to note that unlike IL-17RD, other IL-17R receptor family members including IL-17RA, IL-17RC and IL-17RE contain a proline and not threonine and this may contribute to the specificity of IL-17RD in negatively regulating TLR signalling. We then investigated the regulatory process by which IL-17RD is triggered to inhibit the recruitment of TRAF6 by MyD88. Human PBMCs were treated with LPS for indicated time points and cell lysates were immunoprecipitated for endogenous IL-17RD and the interaction of MyD88 assessed. LPS caused a time-dependent interaction of IL-17RD with MyD88 ( Fig. 6a ). We finally assessed whether we could detect endogenous complexes of IL-17RD and MyD88 in situ and employed a proximity ligation assay for this purpose. While these complexes were not apparent in unstimulated PBMCs, LPS was shown to promote formation of endogenous complexes of IL-17RD and MyD88 in situ in PBMCs ( Fig. 6b ). It is of interest to note that neither the co-immunoprecipitation or proximity ligation assay showed any detectable basal interaction of endogenous IL-17RD with MyD88, suggesting that the interaction is dependent on TLR4 signalling triggering some mechanism to facilitate the interaction. This is also consistent with our inability to detect any in vitro interaction of recombinant forms of IL-17RD and MyD88 ( Supplementary Fig. 6 ). Overall, these data suggest a new autoregulatory network for controlling and terminating TLR signalling pathways. The engagement of TLRs by respective ligands results in the recruitment of TIR adaptors to the receptor complex followed by subsequent recruitment of downstream effectors such as TRAF6. We now propose a model in which this is followed by TLR-induced recruitment of IL-17RD to TIR adaptors thus inhibiting their interaction with their effectors resulting in termination of signalling. 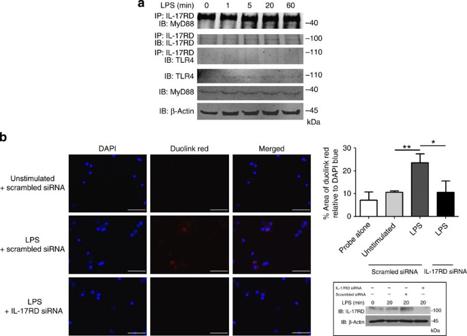Figure 6: LPS inducesin situassociation of IL-17RD with MyD88. (a) PBMCs from human donor blood were treated with LPS (100 ng ml−1) for 0, 1, 5, 20 and 60 min and cell lysates were subject to immunoprecipitation with an anti-IL-17RD antibody. Cell lysate and immunoprecipitate samples were immunoblotted with indicated antibodies. (b) PBMCs from human donor blood were transfected with scrambled or IL-17RD-specific siRNA and cultured for 48 h prior to treatment in the absence or presence of LPS (100 ng ml−1) for 20 min. Cells were fixed to slides and subjected to Duolinkin situproximity ligation assay using anti-IL-17RD and anti-MyD88 antibodies. IL-17RD/MyD88 interactions are visible as red fluorescence of the Duolink detection reagents with nuclear staining in blue (DAPI). Images were captured using the × 20 objective of a fluorescent microscope with scale bars representing 50 μm. The histogram represents the area of red Duolink signal as a percentage of area of blue DAPI signal from five random images from each of three independent experiments. Probe alone indicates areas of signals from cells subjected to ligation assay, but in the absence of anti-IL-17RD and anti-MyD88 antibodies (five random images from each of the two independent experiments). Data are presented as the mean ±s.e.m. and were subjected to a two-tailed paired Student’st-test. *P<0.05; **P<0.01. The lowest-right panel demonstrates knockdown of IL-17RD expression by IL-17RD-specific siRNA as determined by immunoblotting of cell lysates from cells treated with LPS with or without prior transfection with IL-17RD-specific siRNA or a scrambled sequence version of this siRNA. Images have been cropped for presentation. Full-size images are presented inSupplementary Fig. 11. Figure 6: LPS induces in situ association of IL-17RD with MyD88. ( a ) PBMCs from human donor blood were treated with LPS (100 ng ml −1 ) for 0, 1, 5, 20 and 60 min and cell lysates were subject to immunoprecipitation with an anti-IL-17RD antibody. Cell lysate and immunoprecipitate samples were immunoblotted with indicated antibodies. ( b ) PBMCs from human donor blood were transfected with scrambled or IL-17RD-specific siRNA and cultured for 48 h prior to treatment in the absence or presence of LPS (100 ng ml −1 ) for 20 min. Cells were fixed to slides and subjected to Duolink in situ proximity ligation assay using anti-IL-17RD and anti-MyD88 antibodies. IL-17RD/MyD88 interactions are visible as red fluorescence of the Duolink detection reagents with nuclear staining in blue (DAPI). Images were captured using the × 20 objective of a fluorescent microscope with scale bars representing 50 μm. The histogram represents the area of red Duolink signal as a percentage of area of blue DAPI signal from five random images from each of three independent experiments. Probe alone indicates areas of signals from cells subjected to ligation assay, but in the absence of anti-IL-17RD and anti-MyD88 antibodies (five random images from each of the two independent experiments). Data are presented as the mean ±s.e.m. and were subjected to a two-tailed paired Student’s t -test. * P <0.05; ** P <0.01. The lowest-right panel demonstrates knockdown of IL-17RD expression by IL-17RD-specific siRNA as determined by immunoblotting of cell lysates from cells treated with LPS with or without prior transfection with IL-17RD-specific siRNA or a scrambled sequence version of this siRNA. Images have been cropped for presentation. Full-size images are presented in Supplementary Fig. 11 . Full size image While efficient functioning of TLR signalling is associated with effective clearance of invading pathogens by specific tailored immune responses, dysregulation of signalling can lead to chronic inflammatory disease, autoimmunity or sepsis. As a consequence, TLR signalling is subject to multiple levels of regulation. We now describe a new regulatory network that involves the functional interplay of the orphan receptor IL-17RD with TLRs. While members of the IL-17 cytokine family and their receptors have been previously shown to synergize with other cytokines and TLRs to augment the inflammatory response to bacterial and fungal infection, the present study demonstrates for the first time that a member of the IL-17R family can negatively regulate TLR signalling. Currently, IL-17RD is classified as an orphan receptor, given that it has no known ligand. In the event that a ligand(s) is subsequently discovered, it will be especially interesting to assess whether it can regulate TLR signalling. However, even in the absence of an identified ligand the present study demonstrates that TLRs can promote the interaction to IL-17RD with TIR adaptors to temper downstream signalling. Interestingly, a recent study indicated that IL-17RD could inhibit IL-1 and TNF signalling by sequestering the NF-κB subunit p50 in the cytoplasm even after IL-1β- and TNF-α-induced IκB degradation [45] . In addition, a splice variant of IL-17RD was reported to promote ubiquitination of TAK1 and JNK and p38 MAPK activation [46] . However, we show in Il17rd −/− murine primary cells that there is an increase in TLR-induced phosphorylation of IKKs and IκBα, suggesting that IL-17RD targets pro-inflammatory signalling pathways upstream of IκB. In addition, phosphorylation of IRF3 and TBK1, in response to poly(I:C), is also enhanced in Il17rd −/− cells, indicating that IL-17RD can target pathways beyond NFκB. In our model, stimulation of TLRs promote the interaction of IL-17RD with TIR adaptor proteins and the SEFIR domain of IL-17RD is crucial for mediating this interaction. A mutant lacking the SEFIR domain failed to interact with MyD88, Mal and TRIF and loss of this interaction led to diminished inhibitory effects on NF-κB activation. In contract, the SEFIR domain alone was capable of targeting adaptors and manifesting inhibitory effects on downstream signalling. The discovery that the TIR domain of TLRs and IL-1Rs and the SEFIR domain of IL-17Rs are part of a larger domain superfamily highlights the importance of such a motif in innate immune signalling [31] . While a previous report indicated that IL-17R signalling can co-operate in a positive manner with some TLRs [47] , we now propose that the IL-17RD-SEFIR domain negatively regulates TIR domain-containing TLRs, and the region of the IL-17RD-SEFIR domain that corresponds to box 3 of TIR domains is central to this function. It is also noteworthy that mutation of a highly conserved threonine residue in this region abolished the functional effects of the IL-17RD SEFIR domain, and it will be interesting to assess whether this residue is subject to phosphorylation and thus regulation by post-translational modification. Binding of IL-17RD to MyD88 failed to inhibit the adaptor from interacting with TLR4 but prohibited TRAF6 recruitment to the complex, constituting a novel negative regulatory mechanism of TLR signalling. As a consequence, polyubiquitination of TRAF6 was greatly increased in Il17rd −/− macrophages and dendritic cells in response to LPS and poly(I:C). This translated into enhanced downsteam activation of NFκB and IRF3 and induction of pro-inflammatory cytokines that ultimately manifested with Il17rd −/− mice being more susceptible to the lethal effects of LPS and poly(I:C). Such studies emphasize the physiological relevance of IL-17RD in controlling exaggerated inflammatory responses. In addition to elucidating a new regulatory network of TLR signalling and a new function for IL-17RD in innate immunity, our findings also emphasize the intricate cross-talk between innate immune signalling pathways. Recent findings have shown that IKKi and TBK1, key kinases in activating IRFs and regulating type-I IFN expression, regulate IL-17 signalling by directly phosphorylating the adaptor molecule Act1 (refs 48 , 49 ). In addition, IL-17 is produced in response to avian influenza virus and respiratory syncytial virus and synergizes with anti-viral signalling pathways [47] . These discoveries demonstrate the growing complexity of IL-17 signalling and its impact on other signalling pathways. Collectively, our data highlight a key role for IL-17RD in facilitating homeostasis of the innate immune response. IL-17 receptors and TLRs are highly conserved throughout evolution, and high sequence identity among related domains makes it tempting to speculate that they derived from the same ancestral precursor receptor. Given such a scenario, it is plausible that IL-17RD, possibly the most evolutionarily ancient of the IL-17R family [50] , retained the ability to tightly regulate other IL-17 and TLR members. TLRs and their ancestral proteins play key dualist roles as mediators of early development in embryogenesis while also fulfilling seminal roles in mediating innate immunity in adult life. In parallel, IL-17RD now emerges as not only a negative regulator of FGF signalling in early developmental patterning but also as a key modulator of innate immune signalling. This highlights the remarkable exploitation of regulatory networks for diverse purposes at different stages of life. Given its negative role in both IL-17R and TLR signalling, it will be of interest to explore whether dysregulated IL-17RD expression and/or activity contributes to chronic inflammatory disease. Indeed, two separate single-nucleotide polymorphisms have been identified in the Il17rd gene, one which contributes to an increased risk in psoriasis [51] and one with a borderline association with Crohn’s disease [52] . The present study provides the first insight into such potential regulatory effects of IL-17RD in disease. Plasmids and reagents Full-length IL-17RD and IL-17RD ΔC were cloned as previously described [32] . IL-17RD E350A, IL-17RD Y330F, IL-17RD SEFIR T496P, IL-17RD SEFIR K497R, IL-17RD SEFIR L504F and IL-17RD SEFIR T496P/K497R were generated by site-directed mutagenesis using pfu Turbo Thermo Fisher Scientific (Waltham, MA). MyD88 TIR (amino acids 160–296), IL-17RD SEFIR ΔBox1 and IL-17RD SEFIR ΔBox3 were generated using Phusion High-Fidelity DNA polymerase from New England Biolabs (Ipswich, MA). IL-17RA, IL-17RA SEFIR, Act1 SEFIR, IL-17RD SEFIR and mIL-17RD were generated by GenScript. TRAF6 was from Tularik (San Francisco, CA). TK Renilla -luciferase reporter construct (phRL-TK) was from Promega (Madison, WI). The NF-κB-luciferase reporter construct and constructs encoding MyD88 and Mal were gifts from Professor Luke O’Neill (Trinity College Dublin, Ireland). The pFR-luciferase and constructs encoding TLR4, TLR3, TRIF and TRAM were from Professor Andrew Bowie (Trinity College Dublin). The IKKi, TBK1 and IRF3/7 Gal4 reporter constructs were gifts from Professor Kate Fitzgerald (The University of Massachusetts Medical School, Worcester, Massachusetts, USA). LPS was from Enzo Life Sciences (Exeter, UK), poly(I:C), Pam2CSK, Pam3CSK, Zymosan, Flagellin, CLO97 and CpG were from Invivogen (San Diego, CA). Anti-human IL-17RD antibodies used were from R&D systems (Minneapolis, USA) and Phoenix Pharmaceuticals (Burlingame, CA) (1:250 working dilution). Anti-murine IL-17RD antibody (1:250) was from Thermo Fisher Scientific. Anti-phospho IκBα (1:500), anti-phospho IKK (1:1,000), anti-IKK (1:1,000), anti-phospho TBK1 (1:750), anti-TBK1 (1:750), anti-phospho IRF3 (1:750), anti-phospho p38 (1:750), anti-p38 (1:750), anti-phospho ERK (1:750), anti-ERK (1:750), anti-phospho JNK (1:750), anti-JNK (1:750) and anti-Myc antibodies (1:1,000) were from Cell Signalling Technology Inc. (Danvers, MA). The anti-HA antibody (1:500) was from Covance Inc. (NJ, USA). Anti-GST (1:1,000), anti-β-actin (1:8,000) and anti-FLAG (1:2,000) antibodies and the Duolink In Situ Red Starter kit Goat/Rabbit were supplied by Sigma-Aldrich (St Louis, USA). Anti-IκBα (1:500), anti-IRF3 (1:500), anti-TRAF6 (1:500), anti-MyD88 (1:250), anti-TLR4 (1:500), anti-ubiquitin (1:500) and anti-p65 (1:500) antibodies were from Santa Cruz Biotechnology (Santa Cruz, CA). Recombinant human MyD88 was from Novus Biologicals (Littleton, CO) and recombinant human IL-17RD was from Origene (Rockville, MD). Mice IL-17RD-deficient mice were generated by the German Genetrap Consortium using its proprietary technology (clone ID: D065E01) as previously described [32] . Briefly, a gene trap vector was incorporated into the Il17rd gene after the first exon in embryonic stem cells of 129S2/SvPas origin. Embryonic stem cells were microinjected into female mice of C57BL/6 background and heterozygous F1 progeny were intercrossed to obtain Il17rd −/− mice. Il17rd +/− mice were bred to generate age- and sex-matched Il17rd +/+ and Il17rd −/− mice for experiments. Breeding, colony expansion and maintenance were performed in the Bioresource facility of the National University of Ireland (NUI), Maynooth. All animals were housed in individually ventilated cages with high-efficieny particulate air filters. All animal experiments were performed in accordance with the regulations and guidelines of the Irish Department of Health and protocols approved by the Biomedical and Life Sciences Research Ethics committee of NUI Maynooth. Cell culture HEK293 and U373 cells were cultured in Dulbecco’s modified Eagle’s medium supplemented with 10% (v/v) fetal bovine serum (FBS), 100 U ml −1 penicillin and 100 μg ml −1 streptomycin. HEK293 TLR3 cells and HEK293 TLR4 cells were maintained in Blasticidin (Invivogen, 10 μg ml −1 ) or G418 (500 μg ml −1 ), respectively. THP-1 suspension cells were grown in Roswell Park Memorial Institute (RPMI) plus GlutaMAX-I medium (Gibco) supplemented with 10% (v/v) FBS, and penicillin/streptomycin (100 units ml −1 and 0.1 mg ml −1 , respectively). Human PBMCs from healthy volunteers were extracted from buffy coats provided by the Irish Blood Transfusion Service. PBMCs were isolated using the Ficoll-Hypaque isolation technique and plated in complete RPMI 1640 medium. For the preparation of primary MEFs, Il17rd +/− mice were bred to generate Il17rd +/+ and Il17rd −/− embryos. Embryos were dissected from pregnant females at day 13 post coitum. MEFs were isolated by standard procedure and cultured in Dulbecco’s modified Eagle’s medium supplemented with 10% (v/v) FBS for 3 days. To isolate BMDMs or BMDCs, tibias and femurs from Il17rd +/+ and Il17rd −/− mice were removed using a sterile technique and the bone marrow was flushed with fresh medium. To obtain macrophages, cells were plated in medium supplemented with M-CSF (20 ng ml −1 ) and maintained at 37 °C in a humidified atmosphere of 5% CO 2 for 4–6 days. To obtain myeloid dendritic cells, cells were plated in medium supplemented with GM-CSF (10 ng ml −1 ) and maintained at 37 °C in a humidified atmosphere of 5% CO 2 for 6–8 days. Medium was replaced with fresh supplemented media every 3 days. All cells were maintained at 37 °C in a humidified atmosphere of 5% CO 2 . Luciferase reporter assay HEK293 cells were seeded (1.5 × 10 5 cells ml −1 ) in 96-well plates (200 μl per well) for 24 h. Cells were then transfected using Lipofectamine 2000 (Invitrogen), according to the manufacturer’s instruction, with constructs encoding NF-κB-regulated firefly luciferase (80 ng) or pFR firefly luciferase reporter construct (60 ng) with IRF3 (30 ng) or IRF7 (25 ng) (both fused downstream of the yeast Gal4 DNA-binding domain), constitutively expressed TK Renilla -luciferase reporter construct (phRL-TK) (40 ng) (Promega Biosciences) and varying amounts of expression constructs as indicated. Total DNA was kept constant (200 ng per well) using the appropriate empty vector. Cell extracts were generated 24 h post transfection using Reporter Lysis Buffer (Promega Biosciences) and extracts were assayed for firefly luciferase and Renilla -luciferase activity using the Luciferase Assay system (Promega Biosciences) and coelenterazine (0.1 μg ml −1 Insight Biotechnology Ltd.), respectively. Luminescence was monitored with the Glomax microplate luminometer (Promega). Data are presented as fold stimulation of firefly luciferase expression relative to unstimulated cells. For siRNA knockdown studies, HEK293 TLR3 and TLR4 cells were seeded (1.5 × 10 5 cells ml −1 ; 3 ml) in six-well plates and grown for 24 h. Cells were then transfected using Lipofectamine 2000 with siRNA and luciferase constructs for 48 h. Cells were treated as indicated and assayed for luciferase activity. Lentiviral production and transduction HEK 293T cells were seeded (2 × 10 5 cells ml −1 ; 3 ml) in six-well plates and grown for 24 h to ~80% confluency. Cells were transfected using Lipofectamine 2000 (Invitrogen) according to the manufacturer’s instructions with the packaging plasmid pCMV-dR 8.91 (1 μg), envelope plasmid VSV-G (1 μg) and IL-17RD sh-pLKO.1 vector (2 μg) or control shRNA (Sigma-Aldrich): IL-17RD shRNA 5′- CCGGCCAGTCTTGGAGAAATTTGATCTCGAGATCAAATTTCTCCAAGACTGGTTTTTG -3′ (NM_017563.1-1819s1c1). Conditioned medium was changed 24 h post transfection and replaced with fresh growth medium containing 30% (v/v) FBS for a further 24 h. The lentiviral-containing medium was harvested and replenished every 24 h for 72 h. U373 and THP-1 cells, seeded (2 × 10 5 cells ml −1 ; 3 ml) in six-well plates, were transduced with 600 μl lentivirus-containing medium with hexadimethrine bromide (8 μg ml −1 ) and incubated at 37 °C for 24 h prior to positive selection of cells with integrated shRNA constructs with puromycin (8 μg ml −1 ). ELISA and type-I IFN bioassay Primary MEFs and BMDMs were seeded in (2 × 10 5 cells ml −1 ; 1 ml) 12-well plates or in (5 × 10 5 cells ml −1 ; 200 μl) 96-well plates and grown for 24 h. Cells were subsequently stimulated with various ligands for the indicated time points as described in figure legends. Conditioned media was collected from each well and measured for levels of TNF-α, IL-6, RANTES, KC (DuoSet kits (R&D Systems)), IL-12/IL-23 p40 (Biolegend) and IFN-β using the Mesoscale Discovery System and murine type-I IFN by blue sensor cells (Invitrogen) as per the manufacturer’s instructions.HEK293, or U373 and THP-1 cells stably transfected with control or IL-17RD-specific shRNA were seeded (2 × 10 5 cells ml −1 ; 200 μl) in 96-well plates and grown for 24 h. In some experiments cells were transfected, using Lipofectamine, with siRNA targeting IL-17RD (sense sequence: 5′- GGAGCAAACUACAGAGAUGTT -3′) or with scrambled siRNA (sense sequence: 5′- GGACAGAACACUAGAUGAGTT -3′) (20 nM) (Ambion) for 48 h. Cells were subsequently stimulated with various ligands for the indicated time points and conditioned media was collected from each well and measured for levels of TNF-α, IL-6, IL-8, RANTES (DuoSet kits (R&D Systems)) and IP-10 (ELISA development Kit (Peprotech)). PBMCs were seeded (2 × 10 5 cells ml −1 ; 200 μl) in 96-well plates and grown for 24 h prior to transfection with siRNA for 48 h with Lipofectamine 2000 (Invitrogen). Cells were treated as indicated and supernatants were measured for levels of IL-8 (DuoSet kits (R&D Systems)) and IFN-β (Mesoscale Discovery System). TLR-induced death and cytokine production in mice Ten to twelve-week-old male Il17rd +/+ and Il17rd −/− mice were administered with LPS (20 mg kg −1 ) or poly(I:C) (5 mg kg −1 ) by i.p. injection for 16 h. Control mice were injected with endotoxin-free PBS. Mice were sacrificed 16 h post administration and serum was taken for enzyme-linked immunosorbent assay (ELISA) analysis. Spleens were snap-frozen in liquid nitrogen and stored at −80 °C for RNA analysis. Livers were fixed in 10% formalin, paraffin-embedded, sectioned at 5 μm and stained with haematoxylin and eosin. The pathologist (J.J.C.) was blinded to the genetic and i.p. treatment of the mice. Ten to twelve-week-old female Il17rd +/+ and Il17rd −/− mice were administered with LPS (20 mg kg −1 ) or poly(I:C) (0.01 μg per g body weight) with D -GAL (0.7 mg per g body weight) by i.p. injection using PBS and D -GAL as respective controls. Mice were observed and weighed twice daily for the duration of the experiment. Mice that became moribund were considered to have reached the end point of the experiment and were euthanized. Power analysis was used to calculate required sample size based on a Power of 0.9 and probability of 0.05. EMSA BMDMs, MEFs or BMDCs were grown in 90-mm culture dishes for 24 h and were stimulated with LPS (10 or 100 ng ml −1 ) or Poly(I:C) (5 μg ml −1 ), respectively. Nuclear extracts were generated as previously described [51] . Nuclear extracts (5 μg) were incubated with LI-COR IRDye 700-labelled oligonucleotide containing the NF-κB-binding site 5- AGTTGAGGGGACTTTCCCAGGC -3′ (κB site underlined) or IRDye 700-labelled oligonucleotide containing the IFNβ PRD I/III-binding site 5′- GTAAATGACATAGGAAAACTGAAAGGGAGAAGTGAAAGTGG -3′ according to the manufacturer’s instructions. For competitive analysis, a non-labelled oligonucleotide of the same sequence was added to the extracts at room temperature (RT) for 15 min prior to incubation with labelled oligonucleotide. Samples were subjected to electrophoresis on a 4% native polyacrylamide gel for 2 h at 70 V and subsequently analysed, and images captured using the Odyssey Infrared Imaging System (LI-COR Biosciences). Retroviral production and transduction HEK 293T cells were seeded (2 × 10 5 cells ml −1 ; 3 ml) in six-well plates and grown for 24 h to 80% confluency. The cells were transfected using Lipofectamine 2000 (Invitrogen) according to the manufacturer’s instructions, with the packaging vector (1 mg) and MSCV plasmid (1 mg) or MSCV-mIL-17RD (1 mg). The cells were then incubated for an additional 24 h. The retroviral-containing medium was harvested and stored at 20 °C. Fresh growth medium containing 30% (v/v) FBS was added to cells and incubated for another 24 h. The virus-containing medium was again harvested and stored for use. WT MEFs and IL-17RD-deficient MEFs were seeded (3 × 10 5 cells ml −1 ; 6 ml) in 25-cm 2 flasks and grown for 4 h. The growth medium was then removed and replaced with fresh medium containing hexadimethrine bromide (8 mg ml −1 ) and 1 ml retrovirus-containing medium from above. The flasks were incubated at 37 °C for 48 h prior to experiments. Immunoblot analysis BMDMs, MEF cells or U373 cells stably transfected with IL-17RD shRNA or control shRNA (3 × 10 5 cells ml −1 ) were seeded in six-well plates and grown for 24 h. Cells were stimulated with LPS (100 ng ml −1 ) or Poly(I:C) (25 μg ml −1 ) for different time points as indicated in the figure legends. Cells were washed in 1 ml of ice-cold PBS and lysed in 100 μl of NP-40 lysis buffer (50 mM Tris-HCl, pH 7.5, containing 150 mM NaCl, 0.5% (w/v) igepal, 50 mM NaF, 1 mM Na 3 VO 4 , 1 mM dithiothreitol (DTT), 1 mM phenylmethylsulfonyl fluoride (PMSF) and complete protease inhibitor mixture (Roche)). The cell lysates were centrifuged at 12,000 g for 10 min, supernatants were collected and subjected to western blotting using the indicated antibodies. Immunoreactive bands were detected using the Odyssey Infrared Imaging System, according to the instructions of the manufacturer. Co-immunoprecipitation analysis Cells were seeded (2 × 10 5 cells ml −1 ; 3 ml or 10 ml) in six-well plates or 90-mm Petri dishes and transfected, using Lipofectamine 2000, with defined amounts of various expression constructs as described above. Cells were washed with pre-chilled PBS (1 ml) and then lysed with pre-chilled lysis buffer (250 μl) (50 mM HEPES, pH 7.5 containing 1 mM EDTA, 10% (v/v) glycerol, 0.05% (w/v) CHAPS, 0.5% (v/v) Triton-X and 250 mM NaCl, 1 mM Na 3 VO 4 , 1 mM DTT, 1 mM PMSF and complete protease inhibitor mixture (Roche)) for 30 min on a rocker at 4 °C. For co-immunoprecipitations with TLR3 and TLR4, a ‘TLR’ lysis buffer (150 mM NaCl, 50 mM Tris-HCL (pH 7.6), 4 mM EDTA, 1% (w/v) Brij, 0.5% (w/v) n -octyl-β- D -glucoside and 0.5% Triton-X-100 (v/v)) was used. Lysates were centrifuged at 12,000 g for 10 min at 4 °C. Aliquots (50 μl) were retained for immunoblotting while the remaining supernatants were removed to fresh pre-chilled tubes. Samples were incubated overnight with the appropriate antibody (2 μg) at 4 °C with rocking. This was followed by the addition of protein A/G agarose beads (30 μl per sample). Incubations were placed at 4 °C with rocking for 4 h. Immunoprecipitates were collected by centrifugation at 1,000 g for 5 min at 4 °C and the beads were then washed four times with lysis buffer (600 μl) lacking the protease inhibitor mixture. The beads were resuspended in 2 × SDS–polyacrylamide gel electrophoresis (PAGE) sample buffer (40 μl) and incubated for 30 min at RT. Samples were centrifuged at 16,000 g for 2 min, subsequently boiled at 100 °C for 5 min and subjected to immunoblotting. The immunoreactive bands were detected and images captured using Odyssey Infrared Imaging System. TRAF6 polyubiquitination studies Primary BMDMs or BMDCs were seeded in cell culture 90-mm dishes (5 × 10 5 cells ml −1 ; 1 × 10 6 cells ml −1 ) and grown for 24 h. Cells were stimulated with LPS or Poly(I:C) for designated times. Cells were washed in 1 ml of ice-cold PBS and lysed in 200 μl of lysis buffer (50 mM HEPES, pH 7.5 containing 1 mM EDTA, 10% (v/v) glycerol, 0.05% (w/v) CHAPS, 0.5% (v/v) Triton-X and 250 mM NaCl, 1 mM Na 3 VO 4 , 1 mM DTT, 1 mM PMSF and complete protease inhibitor mixture (Roche)). The cell lysates were centrifuged at 12,000 g for 10 min and supernatants were collected. Aliquots (20 μl) of these whole-cell lysates were retained for immunoblotting while the remaining supernatants were treated with 1% SDS and incubated at 95 °C for 5 min to dissociate protein–protein interactions. Samples were then diluted 10-fold with lysis buffer prior to incubation overnight with the indicated antibody (2 μg) at 4 °C with rocking. This was followed by the addition of protein A/G agarose beads (30 μl per sample). Incubations were placed at 4 °C with rocking for 24 h. Immunoprecipitates were collected by centrifugation at 12,000 g for 1 min at 4 °C and the beads were then washed four times with lysis buffer (600 μl) lacking the protease inhibitor mixture. The beads were resuspended in 2 × SDS–PAGE sample buffer (40 μl) and incubated for 20 min at RT. Samples were centrifuged at 12,000 g for 1 min, subsequently boiled at 100 °C for 5 min and subjected to SDS–PAGE and immunoblotting using the indicated antibodies. The immunoreactive bands were detected and images captured using Odyssey Infrared Imaging System or using an enhanced chemiluminescent substrate. In vitro co-immunoprecipitation assay Full-length recombinant human IL-17RD-Myc (1.5 μg) was incubated with full-length recombinant human MyD88-GST (1 μg) for 1 h at 4 °C with rocking in reaction buffer (25 mM Tris-HCl, 100 mM NaCL, 3% (v/v) glycerol, 0.05% (v/v) Triton-X). Samples were then incubated with a specific anti-GST antibody (1 μg) 1 h at 4 °C with rocking. This was followed by the addition of protein A/G agarose beads (30 μl per sample) with rocking for 1 h. Immunoprecipitates were collected by centrifugation at 12,000 g for 1 min at 4 °C and the beads were then washed three times with reaction buffer. Washes were saved and flow-through protein was concentrated using Amicon Ultra filters (0.5 ml) (Millipore). The beads were resuspended in 2 × SDS–PAGE sample buffer (40 μl) and incubated for 20 min at RT. Samples were centrifuged at 12,000 g for 1 min, subsequently boiled at 100 °C for 5 min and subjected to SDS–PAGE and immunoblotting using the indicated antibodies. RNA isolation and quantitative PCR BMDMs, MEFs and U373 cells stably transfected with control or IL-17RD shRNA were seeded (2 × 10 5 cells ml −1 ; 3 ml) into six-well plates and grown for 24 h. Cells were then treated with various ligands for the indicated time points. Cells were washed in PBS and RNA was extracted using Tri-Reagent (Sigma) according to the manufacturer’s instructions. Total RNA was also isolated from spleens, had been snap-frozen in liquid nitrogen and homogenized in 1 ml of Tri-Reagent. After DNase I digestion, complementary DNA was generated from normalized RNA using AMV reverse transcriptase (Promega). Samples were assayed by quantitative real-time PCR using Brilliant SYBR Green QPCR Master mix (Stratagene). For the amplification of the specific genes, the following primers were used: hIfnb1 forward 5′- GACCAACAAGTGTCTCCTCCAAA -3′ and reverse 5′- CTCCTCAGGGATGTCAAAGTTCA -3′; mIfnb1 , forward 5′- GGAGATGACGGAGAAGATGC -3′ and reverse 5′- CCCAGTGCTGGAGAAATTGT -3′; mTnf , forward 5′- CATCTTCTCAAAATTCGAGTGACAA -3′ and reverse 5′- TGGGAGTAGACAAGGTACAACCC -3′; hIl8 , forward 5′- CACCGGAAGGAACCATCTCACTGT -3′ and reverse 5′- TCCTTGGCAAAACTGCACCTTCA -3′; mCxcl1 , forward 5′- AGACCATGGCTGGGATTCAC -3′ and reverse 5′- CAAGGGAGCTTCAGGGTCAA -3′; mIl6 , forward 5′- ACAACCACGGCCTTCCCTAC -3′ and reverse 5′- TCCACGATTTCCCGAGAACA -3′; mCcl5 , forward 5′- GGAGATGAGCTAGGATAGAGGG -3′ and reverse 5′- TGCCCATTTTCCCAGGACCG -3′; hIl17rd , forward 5′- CTGTCTCTGCCACTGATGGA -3′ and reverse 5′- AGAGGAGCTTGGAAGGAAGG -3′; mIl17rd , forward 5′- ACCTGAGCACCAAGTACAAGCTCA -3′ and reverse 5′- TGCAAATGGCAACATACAGGGAGC -3′; mCxcl10 , forward 5′- GACGGTCCGCTGCAACTG -3′ and reverse 5′- GCTTCCCTATGGCCCTCATT -3′; mInos forward 5′- CAAGCACCTTGGAAGAGGAG -3′ and reverse 5′- AAGGCCAAACACAGCATACC -3′; mHprt , forward 5′- GCTTGCTGGTGAAAAGGACCTCTCGAAG -3′ and reverse 5′- CCCTGAAGTACTCATTATAGTCAAGGGCAT -3′; hHprt , forward 5′- AGCTTGCTGGTGAAAAGGAC -3′ and reverse 5′- TTATAGTCAAGGGCATATCC -3′. Confocal microscopy HEK293 TLR4 cells were seeded (2 × 10 5 cells ml −1 ) in four-well chamber slides (Lab-Tek, Nunc A/S, Roskilde, Denmark) and grown for 24 h to 80% confluence. Cells were transfected using Lipofectamine 2000 with plasmids encoding MyD88-pEGFP with IL-17RD-pRFP. Processing of samples was performed on ice. Medium was removed, and the cells were gently washed three times in chilled 1 × PBS (500 μl). Cells were then fixed by the addition of 2% (v/v) paraformaldehyde (500 μl) for 20 min. Cells were washed three times with PBS. Nuclei were stained with an aliquot (500 μl) of 4',6-diamidino-2-phenylindole (DAPI) (1.5 μg ml −1 ; Sigma) for 2 min. Cells were mounted with Vectashield hardset mounting medium (Molecular Probes Inc.). Confocal images were captured using the × 40 or × 63 objective lens on the UV Zeiss 510 Meta System laser scanning microscope equipped with the appropriate filter sets. Acquired images were analysed using the LSM 5 browser imaging software. In situ proximity ligation assay PBMCs were seeded (1 × 10 6 cells ml −1 ; 10 ml) in 90-mm Petri dishes and transfected, using Lipofectamine 2000, with 40 nM of scrambled or IL-17RD-specific siRNA. Cells were adhered to poly-l-lysine (Sigma)-coated microscope slides and fixed using acetone/methanol (1:1) at −20 °C for 10 min. Slides were treated with a blocking buffer (PBS containing 1% (w/v) BSA) for 30 min followed by incubation with goat anti-human IL-17RD (10 μg ml −1 ) (R&D) and rabbit anti-human MyD88 (1:100 dilution) (Enzo) primary antibodies in blocking buffer for 1 h at RT. Slides were then incubated with Duolink PLA Rabbit MINUS and PLA Goat PLUS probes (Sigma) for 1 h at 37 °C in a humidity chamber followed by ligation and amplification steps as described by manufacturers of the Duolink In Situ Red Starter kit Goat/Rabbit (Olink Bioscience, Uppsala, Sweden). Ligations were visible as red fluorescence of the Duolink detection reagents with nuclei staining blue from the DAPI-containing mounting medium. Images were captured using the × 20 objective of a fluorescent microscope. Image analysis was performed using Olympus cellSens Dimension 1.9 software and interactions quantitated as areas of red Duolink signal normalized to areas of blue DAPI signal. Statistical analysis Data are expressed relative to untreated cells and are the means ±s.e.m. of triplicate determinations from three independent experiments. For comparison between two groups, Student’s two-tailed paired t -test was used. For comparison between serum and tissue samples from mice or PBMCs from different donors Student’s two-tailed unpaired t -test was used. The log-rank test was used for survival studies. A P value of <0.05 was considered significant. How to cite this article : Mellett, M. et al . Orphan receptor IL-17RD regulates Toll-like receptor signalling via SEFIR/TIR interactions. Nat. Commun. 6:6669 doi: 10.1038/ncomms7669 (2015).